PI3Kδ inhibition reduces TNF secretion and neuroinflammation in a mouse cerebral stroke model Stroke is a major cause of death worldwide and the leading cause of permanent disability. Although reperfusion is currently used as treatment, the restoration of blood flow following ischaemia elicits a profound inflammatory response mediated by proinflammatory cytokines such as tumour necrosis factor (TNF), exacerbating tissue damage and worsening the outcomes for stroke patients. Phosphoinositide 3-kinase delta (PI3Kδ) controls intracellular TNF trafficking in macrophages and therefore represents a prospective target to limit neuroinflammation. Here we show that PI3Kδ inhibition confers protection in ischaemia/reperfusion models of stroke. In vitro , restoration of glucose supply following an episode of glucose deprivation potentiates TNF secretion from primary microglia—an effect that is sensitive to PI3Kδ inhibition. In vivo , transient middle cerebral artery occlusion and reperfusion in kinase-dead PI3Kδ (p110δ D910A/D910A ) or wild-type mice pre- or post-treated with the PI3Kδ inhibitor CAL-101, leads to reduced TNF levels, decreased leukocyte infiltration, reduced infarct size and improved functional outcome. These data identify PI3Kδ as a potential therapeutic target in ischaemic stroke. Acute occlusion of the cerebral arteries results in immediate loss of oxygen and glucose to the core region of the affected brain tissue. A series of ischaemic cascades is rapidly activated, interfering with endogenous repair mechanisms of the ischaemic brain tissue. To date, there are only three recommended treatments for acute ischaemic stroke—plasminogen activator, aspirin and stroke unit, of which only plasminogen activator restores the blood flow by promoting reperfusion [1] . However, reperfusion is also associated with a strong inflammatory response mediated by proinflammatory cytokines such as tumour necrosis factor α (TNF) [2] , [3] , [4] , [5] . This release of cytokines is accompanied by activation of glial cells, vascular endothelial activation, leukocyte infiltration and neuronal apoptosis [5] , [6] , [7] . Inflammation contributes to tissue damage [8] and has been linked to a worsening of clinical outcomes [9] , [10] . TNF antagonists, which block both soluble and membrane-bound biologically active TNF, have therefore been tested in stroke, albeit with limited success [7] , [11] , [12] . Although the inflammatory response is regarded as harmful in stroke, a low, basal level of TNF in the central nervous system (CNS) is also important for neuronal survival [6] , [13] . Furthermore, strategies aimed at eliminating the soluble form of TNF using inhibitors of TNF-converting enzyme suffer from a lack of specificity [14] . Directly blocking the release of pathogenic TNF, while maintaining homoeostatic pools of TNF, may thus be more effective when aiming to attenuate neuroinflammation following reperfusion therapy in stroke. Phosphoinositide 3-kinase delta (PI3Kδ) regulates inflammatory and oncological processes, and PI3Kδ inhibitors are being explored clinically as pharmacological treatments for inflammatory disease and cancer [15] . PI3Kδ inhibitors have shown remarkable therapeutic impact on phase III (ref. 16 ) trials in chronic lymphocytic leukaemia and non-Hodgkin’s lymphoma [16] , [17] . We have recently shown that PI3Kδ activity regulates post-Golgi transport and secretion of TNF in macrophages [18] , [19] . PI3Kδ is similarly implicated in the release of cytokines from other immune cells [20] , [21] , [22] , [23] , [24] , and PI3Kδ-selective inhibitors have significant anti-inflammatory efficacy [24] , [25] , [26] . A dual PI3Kγ/δ inhibitor has been shown to reduce damage in myocardial infarction [27] . However, despite its putative key role in post-ischaemic inflammation, PI3Kδ has not yet been studied in the context of stroke. Our study highlights a novel role for PI3Kδ in stroke-induced injury. Our results show that PI3Kδ regulates TNF secretion from primary microglia as PI3Kδ inhibition dampens TNF release induced by a protocol of glucose deprivation (GD)/restoration in vitro . Besides, genetic or pharmacological inactivation of PI3Kδ improves ischaemic outcomes in mice, reduces TNF in microglia as early as 3 h post ischaemia and impairs leukocyte recruitment to the injured hemisphere. Our results demonstrate that inactivation of PI3Kδ in the brain, and not in the peripheral immune system, is the key initiator of these protective effects. PI3Kδ mediates TNF secretion in primary microglia In vitro , PI3Kδ is not detectable by immunocytochemistry in astrocytes but is present in neurons [28] and microglia in which it appears concentrated at the perinuclear Golgi [18] ( Fig. 1a ). To identify the principal TNF producers in the brain, we measured TNF secretion from primary microglia, astrocytes and neurons in response to GD, which mimics the hypoglycaemic conditions during stroke [29] ; treatment with lipopolysaccharide (LPS), the prototypical activator of TNF secretion in vitro ; or a combination of both treatments. No significant TNF release was detected in astrocytes or neurons. In contrast, microglia secreted high levels of TNF in response to LPS and to a lesser extent in response to GD ( Fig. 1b ). In keeping with our previous study in macrophages [18] , microglia from PI3Kδ kinase-inactive (p110δ D910A/D910A ) [30] mice secreted significantly less TNF in response to LPS than wild-type controls ( Fig. 2a,b ). Similar observations were made in microglia from wild-type mice that were treated ex vivo with the PI3Kδ-selective inhibitor IC87114 (ref. 18 ) or CAL-101 (ref. 23 ), the latter being a highly specific inhibitor that is 40- to 300-fold more selective for PI3Kδ than other PI3K class I enzymes [31] ( Fig. 2a,b ). Intriguingly, GD dramatically reduced LPS-induced TNF secretion from microglia ( Fig. 1b ), suggesting that glucose removal might impair PI3Kδ-sensitive TNF biosynthesis and/or secretion by these cells ( Fig. 2c,d ). To test this hypothesis, we mimicked the paradigm of reperfusion after stroke by replacing the glucose-free medium with normal glucose-containing culture medium following 1 h GD. Such glucose restoration following 1 h of GD significantly increased TNF secretion, an effect that could be blocked by PI3Kδ inhibition ( Fig. 3a ). Using an assay to assess the intracellular trafficking of TNF [18] , [32] , we found that TNF surface delivery was enhanced under conditions of glucose restoration, in a PI3Kδ-sensitive manner ( Fig. 3b ). Intracellular TNF levels remained unchanged after 1 h of GD (followed by 5 h glucose restoration) in p110δ D910A/D910A -derived or CAL-101-treated wild-type microglia ( Fig. 3c ), suggesting that the de novo synthesis of TNF was not altered. Taken together, these data demonstrate that PI3Kδ activity is required for TNF trafficking and secretion on glucose restoration following GD in microglia. 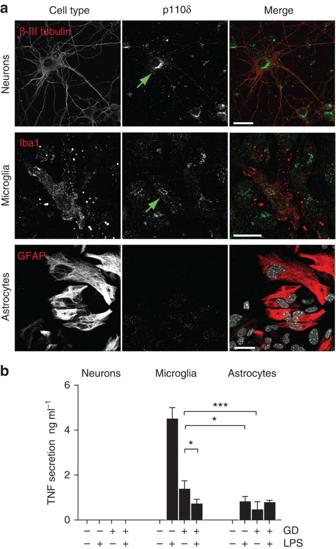Figure 1: PI3Kδ expression and TNF secretion from cortical brain cells. (a) PI3Kδ (green) distributed diffusely through the cytoplasm and in the Golgi region in neurons (βIII-tubulin; red) and microglia (Iba1; red). Little or no PI3Kδ labelling (green channel) was seen in astrocytes (GFAP; red channel). Scale bar, 10 μm. (b) Primary microglia secrete TNF in response to 100 ng ml−1LPS or glucose deprivation (GD). GD or LPS treatment were for 6 h. Data are means±s.e.m.,n=4 cultures. *P<0.05; ***P<0.001; two-tailed Student’st-test. Figure 1: PI3Kδ expression and TNF secretion from cortical brain cells. ( a ) PI3Kδ (green) distributed diffusely through the cytoplasm and in the Golgi region in neurons (βIII-tubulin; red) and microglia (Iba1; red). Little or no PI3Kδ labelling (green channel) was seen in astrocytes (GFAP; red channel). Scale bar, 10 μm. ( b ) Primary microglia secrete TNF in response to 100 ng ml −1 LPS or glucose deprivation (GD). GD or LPS treatment were for 6 h. Data are means±s.e.m., n =4 cultures. * P <0.05; *** P <0.001; two-tailed Student’s t- test. 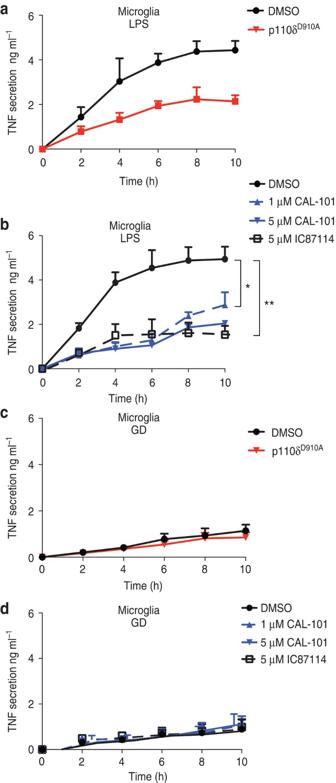Figure 2: Effects of PI3Kδ inhibitors on TNF secretion from LPS-stimulated or glucose-deprived microglia. TNF secretion from wild-type or p110δD910A/D910Aprimary microglia cultures in response to 100 ng ml−1LPS stimulation (a) or GD (b) over a 10-h time course. TNF secretion from wild-type microglia cultures after LPS stimulation (b) or GD (d) in the continuous presence of vehicle dimethylsulphoxide (DMSO), CAL-101 or IC871184 at the indicated concentrations. Data (a–d) are means±s.e.m.,n=3 cultures. *P<0.05; **P<0.01; two-tailed Student’st-test. Full size image Figure 2: Effects of PI3Kδ inhibitors on TNF secretion from LPS-stimulated or glucose-deprived microglia. TNF secretion from wild-type or p110δ D910A/D910A primary microglia cultures in response to 100 ng ml −1 LPS stimulation ( a ) or GD ( b ) over a 10-h time course. TNF secretion from wild-type microglia cultures after LPS stimulation ( b ) or GD ( d ) in the continuous presence of vehicle dimethylsulphoxide (DMSO), CAL-101 or IC871184 at the indicated concentrations. Data ( a – d ) are means±s.e.m., n =3 cultures. * P <0.05; ** P <0.01; two-tailed Student’s t- test. 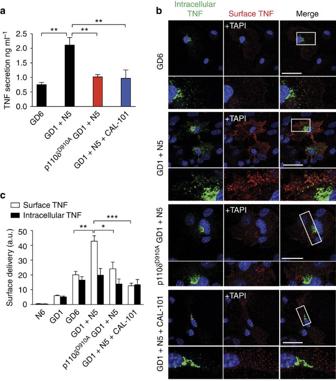Figure 3: PI3Kδ controls TNF trafficking and release elicited by glucose restoration in glucose-deprived microglia. (a) TNF secretion from wild-type microglia cultures (n=5–9) subjected to glucose deprivation (GD) for either 1 h (GD1) or 6 h (GD6) followed by replacement with normal culture medium containing 25 mM glucose for another 5 h (N5) in the continuous presence or absence of CAL-101 (1 μM). (b) Addition of the TNF-converting enzyme (TACE) inhibitor (TAPI), retained TNF at the cell surface for immunostaining (red). Microglia were then permeabilized for intracellular TNF staining (green). 4',6-Diamidino-2-phenylindole (DAPI)-stained nuclei are depicted in blue. Scale bar, 20 μm. (c) Quantification of surface and intracellular TNF staining intensity fromb,n=18–24 cells. Data (a–c) are means±s.e.m. *P<0.05; **P<0.01; ***P<0.001, two-tailed Student’st-test. Full size image Figure 3: PI3Kδ controls TNF trafficking and release elicited by glucose restoration in glucose-deprived microglia. ( a ) TNF secretion from wild-type microglia cultures ( n =5–9) subjected to glucose deprivation (GD) for either 1 h (GD1) or 6 h (GD6) followed by replacement with normal culture medium containing 25 mM glucose for another 5 h (N5) in the continuous presence or absence of CAL-101 (1 μM). ( b ) Addition of the TNF-converting enzyme (TACE) inhibitor (TAPI), retained TNF at the cell surface for immunostaining (red). Microglia were then permeabilized for intracellular TNF staining (green). 4',6-Diamidino-2-phenylindole (DAPI)-stained nuclei are depicted in blue. Scale bar, 20 μm. ( c ) Quantification of surface and intracellular TNF staining intensity from b , n =18–24 cells. Data ( a – c ) are means±s.e.m. * P <0.05; ** P <0.01; *** P <0.001, two-tailed Student’s t- test. Full size image PI3Kδ inhibition protects from ischaemia To recapitulate reperfusion in ischaemic stroke in vivo , we induced transient middle cerebral artery occlusion (tMCAO) [28] , [33] , [34] , [35] in wild-type and p110δ D910A/D910A mice, followed by 24–72 h reperfusion ( Fig. 4a–c ). The extent of brain damage and neurological deficit measured 72 h after ischaemia/reperfusion (I/R) was significantly lower in p110δ D910A/D910A mice than in wild-type mice. Similarly, a single intravenous dose of 40 mg kg −1 of CAL-101, given 15 min before ischaemia in wild-type mice (pre-treatment), significantly reduced infarction after 72 h ( Fig. 4d,e ). However, lower doses (20, 10 and 1 mg kg −1 ) did not achieve significant protection ( Fig. 4e ). Importantly, even when given 3 h after the onset of reperfusion (post-treatment), a dose of 40 mg CAL-101 per kg body weight was still effective in reducing the infarct volume by an average of 44% compared with the vehicle-treated control group. Pre- or post-treatment (3 h) with CAL-101 also consistently improved neurological scores following tMCAO ( Fig. 4f ). The benefits of CAL-101 treatment on stroke outcomes were no longer evident if the drug was administered 6 h after I/R, with infarct sizes not significantly different from those observed in vehicle-treated mice (44.05±4.16% versus 45.91±4.30%, respectively, n =6). PI3Kδ inhibition thus protects against reperfusion-induced damage in the brain for up to at least 3 h after an ischaemic insult. 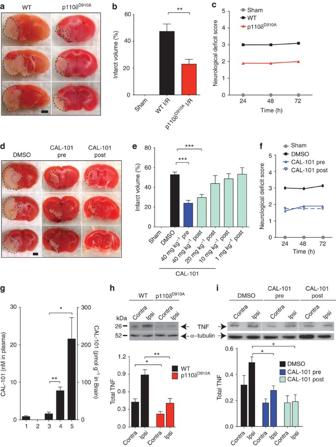Figure 4: Genetic or pharmacological inhibition of PI3Kδ reduces cerebral infarction and improves neurological outcome in ischaemia/reperfusion (I/R). Representative images (a) and graph (b) of infarct volume measurements in wild-type (WT) and p110δD910A/D910Amice subjected to transient middle cerebral artery occlusion (tMCAO) for 1 h followed by 72 h reperfusion. Scale bar, 2 mm. (c) Neurological scores evaluated at 24, 48 and 72 h (n=8–23 mice per group) based on a five-point system: 0, no deficit; 1, failure to extend right paw; 2, circling to the right; 3, falling to the right; and 4, unable to walk spontaneously. (d) Representative images of infarct volumes in wild-type mice treated with vehicle dimethylsulphoxide (DMSO) or CAL-101 (40 mg kg−1i.v.) 15 min before ischaemia (Pre) or 3 h after reperfusion (Post). Scale bars, 2 mm. (e) Graph depicting infarct volume measurements in wild-type mice treated i.v. with DMSO or CAL-101 at the indicated concentrations. Infarct volume data are %±s.e.m (relative to total contralateral hemisphere),n=7–28 mice per group. **P<0.01; ***P<0.001, one-way analysis of variance (ANOVA) and Turkey’spost hoctest. (f) Neurological deficit scores at indicated times post-tMCAO in wild-type mice treated with DMSO or CAL-101 (40 mg kg−1i.v.) 15 min before ischaemia (CAL-101 Pre) or 3 h after reperfusion (Post). (g) Plasma (nmol l−1) and brain (pmol g−1) concentrations of CAL-101 in mice measured by LC- MS/MS: (1) sham+CAL-101 (plasma), (2) sham−CAL-101 (brain), (3) sham+CAL-101 (brain), (4) I/R+CAL-101 3 h post treatment (perfused brain), (5) I/R+CAL-101 3 h post treatment (non-perfused brain); data are mean±s.e.m,n=3 mice per group. *P<0.05; **P<0.005. (h) Western blot of the contralateral and ipsilateral hemispheres of wild-type and p110δD910A/D910Abrains after 24 h I/R. Densitometric measurements (mean±s.e.m.) of TNF normalized to tubulin,n=4 mice per group. *P<0.05; **P<0.01, two-tailed Student’st-test. (i) Western blot of the contralateral and ipsilateral hemispheres of DMSO- and CAL-101-treated mice after 24 h I/R. Densitometric measurements (mean±s.e.m.) of TNF normalized to α-tubulin,n=4 mice per group. *P<0.05, two-tailed Student’st-test. Figure 4: Genetic or pharmacological inhibition of PI3Kδ reduces cerebral infarction and improves neurological outcome in ischaemia/reperfusion (I/R). Representative images ( a ) and graph ( b ) of infarct volume measurements in wild-type (WT) and p110δ D910A/D910A mice subjected to transient middle cerebral artery occlusion (tMCAO) for 1 h followed by 72 h reperfusion. Scale bar, 2 mm. ( c ) Neurological scores evaluated at 24, 48 and 72 h ( n =8–23 mice per group) based on a five-point system: 0, no deficit; 1, failure to extend right paw; 2, circling to the right; 3, falling to the right; and 4, unable to walk spontaneously. ( d ) Representative images of infarct volumes in wild-type mice treated with vehicle dimethylsulphoxide (DMSO) or CAL-101 (40 mg kg −1 i.v.) 15 min before ischaemia (Pre) or 3 h after reperfusion (Post). Scale bars, 2 mm. ( e ) Graph depicting infarct volume measurements in wild-type mice treated i.v. with DMSO or CAL-101 at the indicated concentrations. Infarct volume data are %±s.e.m (relative to total contralateral hemisphere), n =7–28 mice per group. ** P< 0.01; *** P <0.001, one-way analysis of variance (ANOVA) and Turkey’s post hoc test. ( f ) Neurological deficit scores at indicated times post-tMCAO in wild-type mice treated with DMSO or CAL-101 (40 mg kg −1 i.v.) 15 min before ischaemia (CAL-101 Pre) or 3 h after reperfusion (Post). ( g ) Plasma (nmol l −1 ) and brain (pmol g −1 ) concentrations of CAL-101 in mice measured by LC- MS/MS: (1) sham+CAL-101 (plasma), (2) sham−CAL-101 (brain), (3) sham+CAL-101 (brain), (4) I/R+CAL-101 3 h post treatment (perfused brain), (5) I/R+CAL-101 3 h post treatment (non-perfused brain); data are mean±s.e.m, n =3 mice per group. * P< 0.05; ** P <0.005. ( h ) Western blot of the contralateral and ipsilateral hemispheres of wild-type and p110δ D910A/D910A brains after 24 h I/R. Densitometric measurements (mean±s.e.m.) of TNF normalized to tubulin, n =4 mice per group. * P <0.05; ** P <0.01, two-tailed Student’s t -test. ( i ) Western blot of the contralateral and ipsilateral hemispheres of DMSO- and CAL-101-treated mice after 24 h I/R. Densitometric measurements (mean±s.e.m.) of TNF normalized to α-tubulin, n =4 mice per group. * P <0.05, two-tailed Student’s t -test. Full size image We next employed liquid chromatography–electrospray ionization–mass spectrometry to quantitatively assess exposure of the brain to CAL-101 following peripheral (intravenous) injection ( Fig. 4g ). Low levels of CAL-101 could be detected in the brains of sham-operated mice, indicating some ability of the inhibitor to cross the blood–brain barrier. Importantly, CAL-101 levels within the brain were significantly increased 24 h after tMCAO, demonstrating increased penetration and exposure to CAL-101 as a result of I/R-associated blood-brain barrier breakdown. Having established the benefits of PI3Kδ inhibition in ischaemic stroke, we next tested whether these protective effects could be related, at least in part, to a reduction in TNF following I/R in vivo . Brains were recovered 24 h after I/R and homogenized hemispheres were analysed for total TNF levels by western blotting. In wild-type control mice with tMCAO, high levels of TNF could be detected in the ipsilateral hemisphere and, to varying degrees, the contralateral hemisphere, consistent with bilateral inflammation following I/R ( Fig. 4h,i ). In contrast, TNF levels were significantly lower in both hemispheres in p110δ D910A/D910A and CAL-101 pre- or post-treated mice ( Fig. 4h , full blots in Supplementary Fig. 1 ). PI3Kδ inhibition reduces TNF in Iba1-positive brain cells We next used TNF and Iba1 immunohistochemistry to monitor TNF expression in microglia/macrophages at the infarct site and other regions of the brain. The infarct core was defined as the region where microtubule-associated protein-2 (MAP-2) was absent [36] and the penumbra as the MAP-2-positive region that was less than 1 mm away from the infarct core. The equivalent contralateral region was also examined. At 24 h after I/R, TNF was detected in Iba1-positive cells ( Fig. 5a–d ) and, to lesser extent, in glial fibrillary acidic protein (GFAP)-positive astrocytes ( Fig. 6a–d ). Co-localization between TNF and Iba1 or GFAP was analysed using Imaris software to derive Pearson’s correlation coefficients ( r ) [37] , [38] . In brain slices from wild-type mice after I/R, co-labelled Iba1/TNF-positive cells were particularly abundant in the ischaemic penumbra ( Fig. 5a,c ; Supplementary Movie 1 ), consistent with the high inflammatory activity in this region [39] . In slices from p110δ D910A/D910A mice or CAL-101 pre-treated mice after I/R, the correlation coefficient of Iba1/TNF-positive cells was significantly reduced by, on average, 73% in the penumbra and 69% in the contralateral areas. Importantly, slices from wild-type mice treated with CAL-101 3 h after onset of reperfusion also still exhibited a significant reduction in Iba1/TNF-positive cells in both the penumbra and contralateral areas ( Fig. 5c,d ; Supplementary Movie 2 ). These results confirm that PI3Kδ inhibition reduces overall TNF immunoreactivity in Iba1-positive cells in regions both proximal and distal to the infarct core. We also observed fewer GFAP-positive astrocytes that were also positive for TNF in p110δ D910A/D910A mice and CAL-101 pre- or post-treated mice ( Fig. 6b,d ; Supplementary Movies 3,4 ). The fact that PI3Kδ could not be detected in astrocytes in vitro ( Fig. 1a ) may indicate that it does not regulate TNF trafficking in this glial cell type. Lastly, in addition to TNF, other inflammatory cytokines such as the interleukins IL-6 and IL-1β were also decreased in the brains of PI3Kδ mice after I/R ( Fig. 7 , full blots in Supplementary Fig. 1 ). To better appreciate the role of PI3Kδ in inflammatory signalling during the very early phases post ischaemia, we carried out a similar analysis of TNF immunoreactivity at 3 and 12 h post I/R in wild-type and p110δ D910A/D910A mice. At these early time points, the vast majority of Iba1-positive cells are of microglial origin as peripheral inflammatory cells have not yet invaded the brain parenchyma [40] . Importantly, as early as 3 h post reperfusion, the high level of co-localization that is normally detected between TNF and Iba1 in activated microglia/macrophages from the ipsilateral I/R side of the wild-type animals was significantly reduced in the same region of the p110δ D910A/D910A mice ( Fig. 5e ). Similar observations were made at 12 h post IR in both the injured and non-injured hemispheres ( Fig. 5f ), in good agreement with a high level of protection being conferred on these animals. In wild-type mice, TNF immunoreactivity appeared diffusely throughout the cytoplasm of Iba1-positive cells ( Fig. 5g ). In sharp contrast, TNF staining always appeared as a perinuclear speck within the same cells in the brains of p110δ D910A mice. This observation is consistent with the hypothesis that PI3Kδ prevents the release and/or expression of inflammatory TNF in Iba1-positive cells [18] . 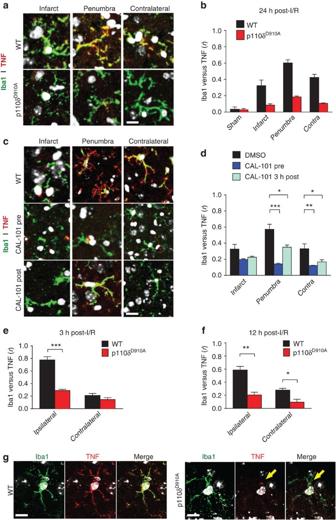Figure 5: Iba1-positive cells with inactive PI3Kδ have reduced TNF immunoreactivityin vivo. Brains from (a) wild-type (WT) or p110δD910A/D910Amice and (c) wild-type mice treated with vehicle dimethylsulphoxide (DMSO) or CAL-101 (40 mg k−1g i.v.) 15 min before ischaemia (CAL-101, Pre) or 3 h after reperfusion (CAL-101, Post) were cryosectioned at 10 μm and analysed for TNF (red) and Iba1 (green) expression in the infarct core, penumbra or contralateral areas (confocal optical sectioning) at 24 h after I/R; cell nuclei are depicted in white. Scale bar, 15 μm. (b,d) Analysis of co-localization of TNF and Iba1 at 24 h post reperfusion, calculated as Pearson’s correlation coefficient,r, on (b) WT versus p110δD910A/D910Amice and (c) wild-type mice treated with vehicle DMSO or CAL-101 (40 mg kg−1i.v.). Data are mean values±s.e.m,n=3 mice per group. (e,f) Wild-type and p110δD910A/D910Amice subjected to transient middle cerebral artery occlusion (tMCAO) for 1 h followed by 3 h (e) to 12 h (f) reperfusion, after which, TNF and Iba1 co-localization was analysed in the ipsilateral (penumbra) and contralateral regions. *P<0.05; **P<0.01; ***P<0.001, two-tailed Student’st-test. (g) Confocal photomicrographs showing a typical Iba1-positive cell in the penumbra of a wild-type and p110δD910Amouse, 3 h after I/R. Note that TNF staining appears throughout the whole Iba1-positive cell in wild-type mice but only as a speck on the periphery of the nucleus in p110δD910Amice (arrow). Scale bar, 15 μm. Figure 5: Iba1-positive cells with inactive PI3Kδ have reduced TNF immunoreactivity in vivo . Brains from ( a ) wild-type (WT) or p110δ D910A/D910A mice and ( c ) wild-type mice treated with vehicle dimethylsulphoxide (DMSO) or CAL-101 (40 mg k −1 g i.v.) 15 min before ischaemia (CAL-101, Pre) or 3 h after reperfusion (CAL-101, Post) were cryosectioned at 10 μm and analysed for TNF (red) and Iba1 (green) expression in the infarct core, penumbra or contralateral areas (confocal optical sectioning) at 24 h after I/R; cell nuclei are depicted in white. Scale bar, 15 μm. ( b , d ) Analysis of co-localization of TNF and Iba1 at 24 h post reperfusion, calculated as Pearson’s correlation coefficient, r , on ( b ) WT versus p110δ D910A/D910A mice and ( c ) wild-type mice treated with vehicle DMSO or CAL-101 (40 mg kg −1 i.v.). Data are mean values±s.e.m, n =3 mice per group. ( e , f ) Wild-type and p110δ D910A/D910A mice subjected to transient middle cerebral artery occlusion (tMCAO) for 1 h followed by 3 h ( e ) to 12 h ( f ) reperfusion, after which, TNF and Iba1 co-localization was analysed in the ipsilateral (penumbra) and contralateral regions. * P <0.05; ** P <0.01; *** P <0.001, two-tailed Student’s t- test. ( g ) Confocal photomicrographs showing a typical Iba1-positive cell in the penumbra of a wild-type and p110δ D910A mouse, 3 h after I/R. Note that TNF staining appears throughout the whole Iba1-positive cell in wild-type mice but only as a speck on the periphery of the nucleus in p110δ D910A mice (arrow). Scale bar, 15 μm. 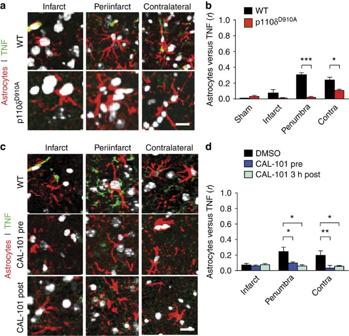Figure 6: Brain astrocytes in PI3Kδ mice have reduced TNF immunoreactivity after 24 h I/R. Brains from (a) wild-type and p110δD910A/D910Amice, or (c) wild-type mice treated with vehicle dimethylsulphoxide (DMSO) or CAL-101 (40 mg kg−1i.v.), 15 min before ischaemia (CAL-101, Pre) or 3 h after reperfusion (CAL-101, Post) were cryosectioned at 10 μm and stained for TNF (red) and GFAP (astrocytes, green). Confocal optical sectioning through the infarct core, penumbra or contralateral areas. Nuclei are depicted in white. Scale bar, 15 μm. (b,d) Analysis of co-localization between TNF and GFAP at 24 h post reperfusion, calculated as Pearson’s correlation coefficient,r. Data are mean values±s.e.m,n=3 mice per group. *P<0.05; **P<0.01; ***P<0.001, two-tailed Student’st-test. Full size image Figure 6: Brain astrocytes in PI3Kδ mice have reduced TNF immunoreactivity after 24 h I/R. Brains from ( a ) wild-type and p110δ D910A/D910A mice, or ( c ) wild-type mice treated with vehicle dimethylsulphoxide (DMSO) or CAL-101 (40 mg kg −1 i.v. ), 15 min before ischaemia (CAL-101, Pre) or 3 h after reperfusion (CAL-101, Post) were cryosectioned at 10 μm and stained for TNF (red) and GFAP (astrocytes, green). Confocal optical sectioning through the infarct core, penumbra or contralateral areas. Nuclei are depicted in white. Scale bar, 15 μm. ( b , d ) Analysis of co-localization between TNF and GFAP at 24 h post reperfusion, calculated as Pearson’s correlation coefficient, r . Data are mean values±s.e.m, n =3 mice per group. * P <0.05; ** P <0.01; *** P <0.001, two-tailed Student’s t- test. 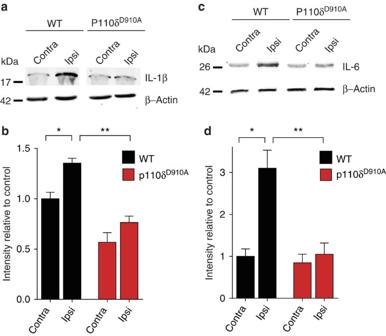Figure 7: Western blot analysis of IL-1β and IL-6 levels in contralateral and ipsilateral hemispheres after 24 h I/R. Representative images (a,b) and densitometric quantification (c,d) of IL-1β (a) and IL-6 (b) protein level normalized to β-actin;n=4 mice per group. Data are represented as mean±s.e.m. *P<0.05; **P<0.01, two-tailed Student’st-test. Full size image Figure 7: Western blot analysis of IL-1β and IL-6 levels in contralateral and ipsilateral hemispheres after 24 h I/R. Representative images ( a , b ) and densitometric quantification ( c , d ) of IL-1β ( a ) and IL-6 ( b ) protein level normalized to β-actin; n =4 mice per group. Data are represented as mean±s.e.m. * P <0.05; ** P <0.01, two-tailed Student’s t -test. Full size image Brain PI3Kδ drives ischaemia-induced leukocyte infiltration To assess the effect of PI3Kδ genetic inactivation or pharmacological inhibition on leukocyte infiltration post reperfusion, analysis of leukocyte populations in the ischaemic hemisphere was carried out with flow cytometry. Twenty-four hours after I/R, p110δ D910A/D910A mice showed a 58% decrease in CD45 high CNS-infiltrating leukocytes in the ipsilesional hemisphere compared with wild-type mice, consistent with reduced inflammation ( Fig. 8a,b ). This protective effect was also achieved with a single, post-treatment dose of CAL-101 administered 3 h after the onset of reperfusion ( Fig. 8d,e ), indicating that inhibition of PI3Kδ after reperfusion is effective in controlling the leukocyte influx into the ischaemic brain. Within the CD45 high infiltrating cell population, we observed a significant reduction in the CD11b + Ly6G + neutrophils from brain homogenates of both p110δ D910A/D910A mice and CAL-101 post-treated mice ( Fig. 8c,f ). 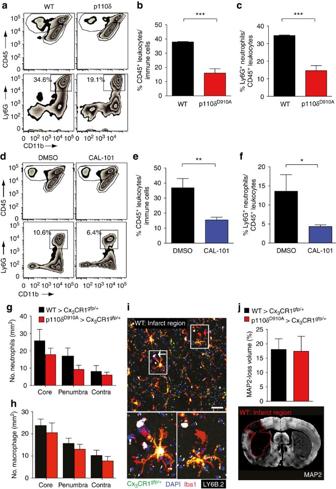Figure 8: Inhibition of PI3Kδ decreases infiltration of CD45+leukocytes in the ischaemic brain 24 h after I/R. Cells recovered on a Percoll gradient from homogenized ipsilesional hemispheres of (a–c) wild-type or p110δD910A/D910Amice (n=4 mice per genotype) or (d–f) wild-type mice treated with vehicle dimethylsulphoxide (DMSO) or CAL-101 (40 mg kg−1i.v.) 3 h after I/R (n=8 mice per group). (a,d) Top: representative contour plots showing gating strategy for CD45highCNS-infiltrating leukocytes and CD45intermediatemicroglia. Bottom: representative contour plots showing CD11b+Ly6G+CNS-infiltrating neutrophils. (b,e) CD45highCNS-infiltrating leukocytes expressed as a percentage of the total immune cells. (c,f) Proportion of neutrophils within the infiltrating CD45highleukocyte population. All flow cytometry data are presented as %±s.e.m. *P<0.05; **P<0.01; ***P<0.001, two-tailed Student’st-test. (g,h) Quantitative cell counts of infiltrating neutrophils and monocytes/macrophages in infarcted brain tissue (1 h of ischaemia and 24 h of reperfusion) of bone marrow (BM) chimeric mice with select deficiency of PI3Kδ within the peripheral immune compartment (p110δD910A/D910A>Cx3cr1gfp/+) and controls (WT>Cx3cr1gfp/+). Data are mean±s.e.m.n=6–8 mice per group. (i) Representative confocal images of neutrophils (white arrow), microglia (green arrow) and infiltrating monocytes/macrophages (red arrow) in the ischaemic infarct zone of BM chimeric mice. Scale bar, 30 μm. (j) Top: infarct volumes in WT>Cx3cr1gfp/+and p110δD910A/D910A>Cx3cr1gfp/+BM chimeric mice; volume is relative to total contralateral hemisphere. Data are %±s.e.m,n=6–8 mice per group. Bottom: representative image showing infarct boundaries as assessed by MAP-2 staining. Figure 8: Inhibition of PI3Kδ decreases infiltration of CD45 + leukocytes in the ischaemic brain 24 h after I/R. Cells recovered on a Percoll gradient from homogenized ipsilesional hemispheres of ( a – c ) wild-type or p110δ D910A/D910A mice ( n =4 mice per genotype) or ( d – f ) wild-type mice treated with vehicle dimethylsulphoxide (DMSO) or CAL-101 (40 mg kg −1 i.v.) 3 h after I/R ( n =8 mice per group). ( a , d ) Top: representative contour plots showing gating strategy for CD45 high CNS-infiltrating leukocytes and CD45 intermediate microglia. Bottom: representative contour plots showing CD11b + Ly6G + CNS-infiltrating neutrophils. ( b , e ) CD45 high CNS-infiltrating leukocytes expressed as a percentage of the total immune cells. ( c , f ) Proportion of neutrophils within the infiltrating CD45 high leukocyte population. All flow cytometry data are presented as %±s.e.m. * P <0.05; ** P <0.01; *** P <0.001, two-tailed Student’s t -test. ( g , h ) Quantitative cell counts of infiltrating neutrophils and monocytes/macrophages in infarcted brain tissue (1 h of ischaemia and 24 h of reperfusion) of bone marrow (BM) chimeric mice with select deficiency of PI3Kδ within the peripheral immune compartment (p110δ D910A/D910A >Cx 3 cr1 gfp/+ ) and controls (WT>Cx 3 cr1 gfp/+ ). Data are mean±s.e.m. n =6–8 mice per group. ( i ) Representative confocal images of neutrophils (white arrow), microglia (green arrow) and infiltrating monocytes/macrophages (red arrow) in the ischaemic infarct zone of BM chimeric mice. Scale bar, 30 μm. ( j ) Top: infarct volumes in WT>Cx 3 cr1 gfp/+ and p110δ D910A/D910A >Cx 3 cr1 gfp/+ BM chimeric mice; volume is relative to total contralateral hemisphere. Data are %±s.e.m, n =6–8 mice per group. Bottom: representative image showing infarct boundaries as assessed by MAP-2 staining. Full size image We next tested whether this diminished infiltration resulted from PI3Kδ inactivation in the CNS or in circulating leukocytes. We used bone marrow (BM) chimera approaches to selectively introduce the p110δ D910A/D910A mutation into the peripheral immune compartment only, which allowed us to specifically examine the role of PI3Kδ in leukocyte recruitment following tMCAO. Transplantation of p110δ D910A/D910A BM into conditioned Cx 3 cr1 gfp/+ hosts revealed no significant differences in neutrophil numbers (Ly6B.2 + Iba1 − GFP − cells) within the infarcted brain tissue at 24 h after I/R compared with controls that received wild-type BM transplants ( Fig. 8g ). The use of Cx 3 cr1 gfp/+ mice as recipient hosts also allowed us to unequivocally distinguish brain microglia (Iba1 + GFP + cells) from infiltrating donor BM-derived monocytes/macrophages (Iba1 + GFP − cells; Fig. 8i ). Taking advantage of this during quantitative image analysis, we also found no differences in the number of infiltrating monocytes/macrophages between experimental groups ( Fig. 8h ), indicating that the lack of PI3Kδ activity in these cells did not negatively affect their recruitment. Infarct size ( Fig. 8j ) was also not different between the experimental groups. Collectively, these findings suggest that a lack of PI3Kδ activity within CNS-resident cells critically contributes towards the protective phenotype observed in p110δ D910A/D910A mice. In this study we reveal a protective effect afforded by inhibiting PI3Kδ in a murine model of stroke. Our data demonstrate that genetic or pharmacological inhibition of PI3Kδ greatly reduces TNF secretion from microglia under ischaemia and reperfusion in vivo or under in vitro GD/restoration. Our data show that inhibition of PI3Kδ up to 3 h post ischaemic stroke has a significant protective effect, and therefore provides an additional therapeutic strategy to be considered in this context. Proinflammatory cytokines such as TNF, IL-1β and IL-6 play multiple roles both in the pathology and recovery after ischaemic brain damage. Microglia activation and TNF release are associated with cell death and pathological inflammation, but they are also implicated in immune tolerance and brain repair. Removing TNF may not be fully beneficial, as this strategy has only had limited success [7] , [11] , [12] , [13] , [14] and TNF-deficient mice appear to have exacerbated cortical infarction and behavioural deficit [41] . One of the underlying reasons may be that a reduction in the homoeostatic levels of TNF may affect neuronal survival [6] , [12] . Consequently, approaches designed to dampen TNF release from microglia or to administer short-lived anti-TNF agents during the acute phase might prove more effective. We have previously demonstrated that PI3Kδ regulates post-Golgi trafficking and secretion of TNF in macrophages stimulated by LPS [18] . Interestingly, PI3Kδ inhibition does not fully abolish TNF secretion under GD conditions in microglia or after tMCAO in mice, supporting the existence of two parallel pathways for TNF secretion: a constitutive low capacity one, independent of PI3Kδ and an inflammation-elicited pathway as previously described [18] , [42] . Difference in cellular sources of TNF might also be important for controlling TNF levels and effects in the brain. Astrocytes also produce and release TNF but they are not sensitive to PI3Kδ inhibition in vitro as they do not exhibit PI3Kδ immunoreactivity, suggesting different trafficking regulators might control TNF release in these cells. The lack of PI3Kδ detection in astrocytes in vitro indicates that the observed decrease in astrocytic TNF in vivo under I/R may result from attenuated proinflammatory feedback cascades [5] , [43] , [44] stemming from reduced microglial TNF secretion. Our study is in good agreement with other studies pointing to a key role of microglial TNF in early-phase inflammation in the CNS [13] . Our in vitro studies also highlight the presence of PI3Kδ in neurons [28] but their role in TNF secretion could not be tested because secreted TNF was not detected by our assay in neuronal cultures exposed to either GD or LPS. The role played by PI3Kδ in neurons will therefore require further investigation. The TNF-mediated inflammatory response is known to lead to an increased permeability of the blood–brain barrier [5] , resulting in leukocyte infiltration. Such leukocytic recruitment following experimental stroke has been documented in several species [45] , [46] . Leukocytes are involved in the secondary progression of brain damage, with a dramatic accumulation of frontline neutrophils occurring in the infarcted tissue during reperfusion [12] , [42] , [47] , an observation replicated in our mouse I/R model. Our results reveal a key role of the PI3Kδ-TNF axis in mediating leukocyte recruitment into the ischaemic brain post reperfusion. TNF can promote the recruitment and migration of CNS-invading leukocytes across the vascular endothelial barrier [48] . Despite this, the BM chimera experiments carried out in our study reveal that the reduced level of leukocyte infiltration detected in the absence of PI3Kδ activity is initiated in the CNS, and does not result from a loss of PI3Kδ in circulating leukocytes. Although the integrity of the blood–brain barrier is known to be greatly altered by stroke, the access of injected inhibitors to the brain is uncertain. Here we provide the first method for the detection of the inhibitor CAL-101 in the brain. Using liquid chromatography–electrospray ionization–mass spectrometry, we confirm the presence of CAL-101 in the brain tissue 24 h after tMCAO. This method is likely to be useful for the detection of CAL-101 in other tissues and for the treatment of other conditions. Taken together, our findings demonstrate that the pharmacological inhibition of PI3Kδ, even post reperfusion, provides organismal protection against reperfusion-induced inflammation in ischaemic stroke, leading to significantly improved neurological outcomes. The efficacy of delayed treatment is highly relevant in a clinical setting for ischaemic stroke. Drugs selectively targeting PI3Kδ can thus potentially be exploited alone or in synergy with existing reperfusion approaches to reduce I/R-induced neuroinflammation. By blocking the intracellular trafficking and secretion of TNF and potentially other proinflammatory cytokines such as IL-1β and IL-6 in Iba1-positive cells, PI3Kδ inhibition represents an attractive strategy to control injurious neuroinflammatory responses within an acute time window in ischaemic stroke. Mice and cerebral focal I/R model p110δ D910A/D910A mice [30] and wild-type littermates bred on a C57BL/6 background were kept under pathogen-free conditions. Blood glucose and haematocrit analyses in male mice revealed no differences between genotypes (blood glucose: 12.40±0.9539 versus 11.60±0.2646, respectively, n =4; haematocrit: 34.38±0.7181 versus 36.50±2.010 n =4), thereby negating a role of these physiological variables in subsequent stroke outcomes. For in vivo experiments with CAL-101, wild-type C57BL/6 mice were used. All animal experiments were approved by the Institutional Animal Ethics Committee and conducted in accordance with the Australian Code of Practice for the care and use of animals for scientific purposes. Mice for all animal experiments were randomized and coded, so experiments were carried out blindly. Exclusion criteria were excessive bleeding or death within 24 h after tMCAO. Male, 12- to 22-week-old, mice were anaesthetized for cerebral focal I/R induction by tMCAO [29] , [33] , [34] , [35] . After a midline neck incision, the left external carotid and pterygopalatine arteries were isolated and ligated with 5-0 silk thread. The internal carotid artery was occluded with a clip at the peripheral site of the bifurcation to the pterygopalatine artery and the common carotid artery was then ligated with 5-0 silk thread. The external carotid artery was cut and a 6-0 nylon suture with a blunted tip (0.20 mm) was inserted. The clip at the internal carotid artery was then removed for advancement of the nylon suture into the middle cerebral artery to slightly more than 6 mm from the internal carotid–pterygopalatine artery bifurcation. After 1 h occlusion, the nylon suture and the ligatures were removed to initiate reperfusion for 24 h up to 72 h. In the sham group, these arteries were visualized but not disturbed. For CAL-101 treatment, wild-type C57BL/6 mice were administered either 40 mg kg −1 CAL-101 (Active Biochem, #A-1138) or vehicle dimethylsulphoxide (Sigma), by 25 μl infusion into the femoral vein, 15 min before I/R (pre-treatment), or 3 and 6 h after initiation of reperfusion (post-treatment). Controls and animals treated with CAL-101 underwent cerebral blood flow (CBF) measurements using a laser Doppler perfusion monitor (Moor Lab). The CBF measurements obtained immediately before and after MCAO and again at 3 h after reperfusion showed an ~90–95% reduction in the blood flow to the MCAO infarct region, which did not differ between groups. Generation of BM chimeric mice Cx 3 cr1 gfp/+ male recipient mice (6–9 months of age) [49] were sublethally irradiated with two doses of 5 Gy delivered 14 h apart and their immune system rescued via BM transplantation from either wild-type (control) or p110δ D910A/D910A donors, 3–4 h after the second dose of irradiation [50] . In the latter group, expression of the kinase-dead form of PI3Kδ was restricted to the peripheral immune compartment only, thereby allowing for the assessment of leukocyte recruitment following ischaemic stroke. BM chimeric mice were let to recover for 20 weeks before being subjected to tMCAO as detailed above. Blood analysis confirmed the efficiency of the chimerization protocol, with over 95% of circulating white blood cells being of donor BM origin. CBF measurements showed an ~80% decrease in the blood flow to the MCAO infarct region, which did not differ between groups. Infarct measurement and neurological assessment Brains from mice euthanized 72 h after I/R were cut into 2 mm coronal sections, before staining with 2% 2,3,5-triphenyltetrazolium chloride (Sigma) in PBS (Sigma) at 37 °C. Infarct sizes were determined from digitized images by measuring the area of damaged tissue in the left (ipsilateral) hemisphere in every section using ImageJ software (version 1.44; NIH) and normalized to the total area of the contralateral hemisphere. After I/R, each mouse was scored every day until the killing on a five-point system [34] , [35] : 0, no neurological deficits; 1, failure to extend right paw; 2, circling to the right; 3, falling to the right; and 4, unable to walk spontaneously. Tissue sections and immunohistochemistry Mice were anaesthetized and transcardially perfused with saline and 10% phosphate-buffered formaldehyde (Sigma). Whole brains were then fixed in 4% paraformaldehyde (Sigma) overnight at 4 °C before sequentially immersing them into 20 and 30% solutions of sucrose (w/v) at 4 °C. For cryosections, the brains were embedded and frozen in TissueTek (Sakura) before being sectioned in the coronal anatomical plane into 10 μm sections using a Microm HM560MV cryostat (Thermo Scientific) and mounted onto glass slides. For antigen retrieval of Iba1 and TNF, sections were treated with 20 μg ml −1 proteinase K (Roche) in 10 mM Tris–HCl (Sigma), pH 7.4. Selected sections were incubated for 1 h in blocking buffer (PBS containing 10% fetal bovine serum (FBS; Life Technologies) and 0.1% Triton X-100 (Sigma)) before primary incubation for 1.5 h with goat anti-Iba1 (Abcam ab5076, 1:100) or rabbit anti-GFAP (Abcam ab7260, 1:500) and mouse anti-TNF (Abcam ab1793, 1:100) diluted in PBS. After washes in 0.1% Triton X-100/PBS for 15 min, the sections were incubated for 1 h with Alexa Fluor488 rabbit anti-goat IgG and Alexa Fluor568 rabbit anti-mouse IgG, or Alexa Fluor568 goat anti-rabbit and Alexa Fluor488 goat anti-mouse (all from Invitrogen, 1:500) diluted in blocking buffer. All incubations were performed at room temperature. After washes in 0.1% Triton X-100/PBS, the slides were counterstained with 4',6-diamidino-2-phenylindole and mounted in Vectashield (Vector Laboratories). Z-series through the coronal sections, 5–9.8 μm in the infarct or penumbra regions to 9.8 μm in the contralateral regions were captured on an inverted confocal microscope (LSM510; Carl Zeiss) with a × 20 (numerical aperture 0.75) objective using the associated ZEN software. LSM images were analysed in Imaris Coloc (version 7.2.3; Bitplane) and Pearson’s correlation coefficient ( r ) values were calculated to measure the correlation dependency of co-localized voxels in three dimension between separate colour channels [37] , [38] . For experiments in BM chimeric mice, brains were cut into 40 μm coronal sections with a microtome (1:4 series) and subjected to free-floating immunofluorescence staining. Mouse anti-MAP-2 (Millipore MAB3418, 1:1,000) staining was used to determine infarct size. For this, an average of 15 free-floating sections were stained per brain and imaged using a Zeiss fluorescence slide scanner, after which infarct sizes were determined by measuring the area of damaged (that is, MAP-2 negative) tissue in the ipsilateral hemisphere, normalizing it to the total area of the contralateral hemisphere. For quantitative assessment of neutrophils as well as infiltrating and microglia-derived macrophage numbers, a separate series of sections was stained with rat anti-Ly6B.2 (AbD Serotec MCA771GA, 1:400) and goat anti-Iba1 (Abcam ab5076, 1:100). Ly6B.2 + Iba1 − neutrophils were counted under the × 20 objective; the number of infiltrating donor BM-derived macrophages was determined by counting the number of Iba1 + GFP − cells on images taken under the × 10 objective of a Zeiss microscope using ApoTome. Immunocytochemistry Neurons or glial cells cultured on coverslips were fixed in 4% paraformaldehyde for staining [18] . Washes were performed in PBS with or without BSA (Sigma) for blocking. Cells were permeabilized in 0.1% Triton X-100/PBS for 5 min before incubation for 1 h with rabbit anti-PI3Kδ antibody (Abcam ab1678, 1:400) [51] and mouse anti-βIII-tubulin (Covance MMS-435P, 1:1,000), goat anti-Iba1 (Abcam ab5076, 1:500) or chicken anti-GFAP (Abcam ab4674, 1:1,000), followed by incubation for 40 min with Cy3-conjugated donkey anti-rabbit antibody and Alexa Fluor488-conjugated donkey anti-mouse, anti-goat or anti-chicken antibody (Invitrogen, 1:500). All antibodies were diluted in blocking buffer. Coverslips were mounted in ProLong gold reagent (Invitrogen). Confocal images were acquired on the LSM510 microscope with a × 63 (numerical aperture 1.4) objective using the ZEN software. Western blotting Whole brains removed from perfused mice 24 h after I/R were immediately dissected into two hemispheres and homogenized in ice-cold tissue buffer (Thermo Scientific) containing protease and phosphatase inhibitors (Roche) before centrifugation at 14,000 r.p.m. for 10 min at 4 °C. The supernatants were then assessed for protein concentration (Bradford assay; Bio-Rad Laboratories), before SDS–polyacrylamide gel electrophoretic protein separation on 10% acrylamide gels. The proteins were transferred to nitrocellulose membranes and incubated with the different antibodies according to the manufacturer’s instructions (TNF, Calbiochem #654300, 1:1,000; IL-1β, Abcam ab5076, 1:500; IL-6, AbD Serotec #AAM15G, 1:500). The membranes were washed, incubated with horseradish peroxidase-conjugated secondary antibodies for 2 h, washed and then exposed to substrate for enhanced chemiluminescence (Pierce Endogen, USA) for 2 min. The signals were visualized using X-ray films (Fujifilm Corporation, Tokyo, Japan). The films were scanned and densitometric analysis was carried out with NIH Image J software. Alternatively, the membranes were incubated with goat anti-rabbit DyLight 800 or goat anti-mouse DyLight 680B (both 1:10,000) and scanned using the Odyssey Infrared Imaging System (LI-COR Biosciences). Primary cortical neurons, astrocytes or microglia Brain cortices were removed from embryonic day 18 mouse embryos (for neuronal cultures) or postnatal day 1 mice (for astrocytes or microglia cultures) [34] . The cortical tissue was incubated in Ca 2+ -/Mg 2+ -free Hank’s balanced salt solution (Thermo Scientific) containing 1 mg ml −1 trypsin (Sigma) for 10 min at 37 °C. The dissociated tissue was then passed through culture medium, which was either Neurobasal medium (Life Technologies) supplemented with B-27 (Life Technologies) and 1% L -glutamine (v/v) for neuronal enrichment, or DMEM (Life Technologies) containing 50% F12 (v/v; Life Technologies), 10% heat-inactivated FBS (Life Technologies) and 1% L -glutamine for glial enrichment. Cells were dissociated by trituration and seeded in either Neurobasal/B-27/ L -glutamine or DMEM:F12/FCS/ L -glutamine medium at densities from 10 5 cells ml −1 (for neurons) to 1.5 × 10 6 cells ml −1 (for glia) [52] . All cells were maintained at 37 °C in humidified 5% CO 2 /95% air. Neurons were cultured for 7 days before experiments, whereas glia-enriched cultures were maintained for 20–25 days, with the medium being replaced every 3–5 days. To harvest microglia, >90% confluent glia cultures were rinsed with FBS-free DMEM:F12 and incubated with 0.05% trypsin for 20 min. Microglia remained adherent, whereas other glial types lifted away [52] . To harvest astrocytes, >70% confluent glia cultures were incubated with 0.25% trypsin for 2 min. Astrocytes were harvested from supernatants. All cells were then plated for experiments. Cell treatments For LPS stimulation, astrocytes or microglia were incubated with 100 ng ml −1 LPS (from Salmonella minnesota Re595; Sigma). For GD experiments, glucose-free Locke’s buffer containing 154 mM NaCl, 5.6 mM KCl, 2.3 mM CaCl 2 , 1 mM MgCl 2 , 3.6 mM NaHCO 3 and 5 mM HEPES, pH 7.2, was used. For drug treatments, cells were incubated with IC87114 (Symansis), CAL-101 (Active Biochem, #A-1138) and LPS, glucose-free Locke’s buffer (GD), or a combination thereof. For TNF surface delivery assay [18] , [32] , TNF-converting enzyme inhibitor was added at the same time as LPS or included in the glucose-free Locke’s buffer (GD). All inhibitors were reconstituted in dimethylsulphoxide (Sigma) with final concentrations <0.1% in assays. Assaying TNF secretion To determine the levels of secreted TNF, a commercial BD OptEIA TNF Elisa Set II (#558534) kit (BD Biosciences) was used to quantify cytokine concentration in samples according to the manufacturer’s instructions. Tandem mass spectrometry Whole-brain samples ( ca. 500 mg) were homogenized in a tissue blender (2 min) in ice-cold 0.32 M sucrose (5 ml). Brain homogenate (100 μl) or plasma (10 μl) was extracted in 10 volumes of acetonitrile/formic acid (99:1, v/v), and centrifuged (13,000 × g , 15 min, 4 °C) to remove precipitated proteins. The clear supernatant was decanted and diluted 1/10 with 2% formic acid (v/v). Sample clean-up was achieved using cation-exchange solid-phase extraction cartridges (Waters Oasis MCX 30 μm 10 mg 1 cc), which provided excellent recoveries (>95% from brain and >99% plasma). The cartridges were pre-conditioned with methanol (1 ml) followed by water (1 ml), and then loaded with the diluted extracts by gravity, and subsequently washed with 2% formic acid (v/v), followed by methanol (1 ml). CAL-101 was eluted using 1 ml of 5% ammonium hydroxide in methanol (v/v). The samples were evaporated using a vacuum concentrator (37 °C, 2 h) and reconstituted in acetonitrile/water 1:1 (50 μl, v/v) containing reserpine (0.05 μM, internal standard). CAL-101 levels were measured by tandem mass spectrometry on a 5500 QTRAP mass spectrometer with TurboV ion source (AB Sciex), connected to a Nexera UHPLC (Shimadzu). Data acquisition and analysis was performed using AB Sciex Analyst 1.5.2 software. The instrument was operated in the positive ion mode under multiple reaction monitoring conditions ( m/z 416.2>176.0 for CAL-101, and m/z 609.2>195.1 for reserpine) using the following parameters: gas heater temperature (400 °C), electrospray gas (20 psi), curtain gas (30 psi), ion spray voltage (5,000 V), declustering potential (80 V), collision energy (45 V) and cell exit potential (10 V). CAL-101 and reserpine eluted at 0.7 min using a linear gradient increasing from 50 to 90% A at 400 μl min −1 over 4 min (HILIC Kinetex column, 75 × 2.1 mm 2 , 2.6 μm, from Phenomenex), using 0.1% formic acid as buffer A, and acetonitrile/water 9:1 (v/v) with 0.1% formic acid as solvent B (injection volume, 5 μl). The lower limits of quantification (as defined by signal/noise ratio ≥10) for CAL-101 were 1 nmol l −1 (plasma, coefficient of variation (CV) 3%, n =3) and 10 pmol g −1 (brain, CV 4%, n =3). Flow cytometry Animals were euthanized and perfused with PBS. Brains were dissected, cerebella were removed and left ischaemic (ipsilesional) hemispheres were selected. Three hemispheres were pooled, digested for 30 min at 37 °C (1 mg ml −1 collagenase, 0.1 mg ml −1 DNAseI in DMEM) and pressed through a cell strainer (40 μm; BD Biosciences). Cells were incubated with standard erythrocyte lysis buffer on ice, separated from myelin and debris by Percoll gradient (GE Healthcare #17-5445-01) centrifugation, and incubated with the following antibody cocktail for 30 min at room temperature in fluorescence-activated cell sorter buffer (0.5% BSA, 0.02% sodium azide in PBS)—CD45 (30-F11, eBioscience #25-0451-82, 1:100), Ly6G (1A8, BD Biosciences #560603, 1:100), CD11b (M1/70, BD #557396, 1:300) [33] . Data were acquired with a LSR II FACS system (BD Biosciences) and analysed with FlowJo (TreeStar). Doublets were excluded with forward scatter (FSC)-A and FSC-H linearity. Statistical analysis Statistical analysis was performed by Student’s t -test or by one-way analysis of variance and Turkey’s post hoc test, as indicated, using Prism software (version 5; GraphPad Software). The sample sizes were chosen based on previous experience and published reports [18] , [34] , [35] . Differences between groups were considered significant at P <0.05. How to cite this article: Low, P. C. et al. PI3Kδ inhibition reduces TNF secretion and neuroinflammation in a mouse cerebral stroke model. Nat. Commun. 5:3450 doi: 10.1038/ncomms4450 (2014).